Systemic regulation of mammalian ageing and longevity by brain sirtuins The silent information regulator 2 (Sir2) family of NAD + -dependent protein deacetylases and deacylases, called sirtuins, has been implicated to be an evolutionarily conserved regulator of ageing and longevity in yeast, worms and flies over the past decade. However, whether sirtuins are responsible for mammalian ageing and longevity control has been debated intensively because whole-body overexpression of Sirt1, the mammalian orthologue of Sir2, fails to promote longevity in mice [1] . Furthermore, a recent study reported the absence of Sir2-dependent life span extension in worms and flies [2] , adding to this controversy. On the other hand, an increasing number of studies have provided more supportive evidence for the importance of sirtuins for ageing and longevity control in model organisms. Indeed, our recent study has demonstrated that Sirt1 in the hypothalamus regulates mammalian ageing and longevity in mice [3] , providing an important resolution to the current controversy. Moreover, brain sirtuins have also been demonstrated to control several age-associated pathophysiological processes in energy homeostasis, cognitive function, emotion and neurogenesis. Therefore, the manipulation of sirtuin activity and expression in the brain might be a great therapeutic strategy to prevent and treat age-associated disorders and extend our health span. In this review we discuss the various physiological roles of brain sirtuins, their impact on ageing and longevity, and potential therapeutic interventions against age-associated diseases based on targeting sirtuins. 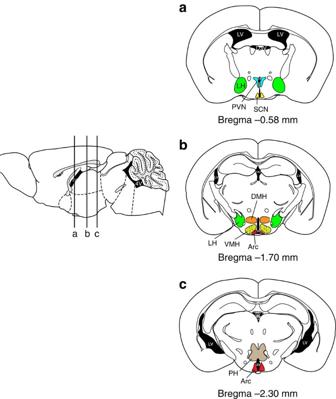Figure 1: Schematic diagrams of brain sections. Sections represent the approximate posterior levels to Bregma −0.58 mm (a), −1.70 mm (b) and −2.30 mm (c). The locations of the hypothalamic nuclei are indicated by the following: LH, lateral hypothalamus; PVN, paraventricular nucleus; SCN, suprachiasmatic nucleus; DMH, dorsomedial hypothalamus; VMH, ventromedial hypothalamus; Arc, arcuate nucleus; PH, posterior hypothalamus. Images adapted, with permission, from Franklin, K.B.J. & Paxinos, G.The Mouse Brain in Stereotaxic Coordinates2nd edn, copyright Academic Press (2001). Various enzymatic activities, cellular localization and physiological functions have been reported for each of the sirtuin family members [4] , [5] , [6] ( Table 1 ). There are seven homologues of sirtuins in mammals, named Sirt1 through Sirt7. Sirt1, Sirt2, Sirt3 and Sirt7 are deacetylases. Sirt5 has been identified to possess deacetylase, desuccinylase and demalonylase activities. Sirt6 has been reported to have deacetylase, ADP-ribosyltransferase, depalmitoylase and demyristoylase activities. Although the enzymatic activity of Sirt4 has not been well characterized, it has at least an ADP-ribosyltransferase activity. For all these enzymatic activities of sirtuins, NAD + is absolutely required [7] , suggesting that sirtuins function as a sensor of the cellular energy status represented by NAD + . Their functions are also compartmentalized in cells. Sirt1, Sirt6 and Sirt7 are mainly localized in the nucleus, whereas Sirt2 is predominantly cytoplasmic. In some cases, both Sirt1 and Sirt2 can shuttle between the nucleus and cytoplasm [5] , [6] . Sirt3, Sirt4 and Sirt5 are localized exclusively in mitochondria. By a number of studies conducted over the last decade, these sirtuin family members have been mainly implicated in the regulation of energy metabolism in a variety of tissues, although they are also involved in many other fundamental biological functions, including DNA repair, cell survival, stress response, telomere and chromatin regulation, autophagy, cancer metabolism, learning and memory, sleep, circadian rhythm and longevity [4] , [5] , [6] . Among these pleiotropic functions of sirtuins, we will focus on their pathophysiological significance in mammalian ageing and longevity control. Table 1 Location, enzymatic activity, interaction partner or target and biological functions of mammalian sirtuins. Full size table The role of sirtuins in the regulation of ageing and longevity was first discovered in Saccharomyces cerevisiae . Yeast mother cells with an extra copy of the Sir2 gene show increases in replicative life span by up to 30%, whereas its deletion or mutation decreases their life span by 50% [6] . This role of Sir2 in life span extension is reproduced by many studies [8] . Moreover, another recent study that uses quantitative trait locus analysis to investigate natural genetic variations associated with longevity in S. cerevisiae further demonstrates that Sir2 plays a critical role in longevity regulation in this organism [9] . Similarly, Caenorhabditis elegans with an increased dosage of sir-2.1, the orthologue of yeast Sir2, shows life span extension by 15–50% [10] . This degree of life span extension in sir-2.1 transgenic worms has been rectified to 10–14% by a recent study [11] after questioning the ability of sir-2.1 to promote longevity [2] . Independent groups also observe sir-2.1-induced life span extension in C. elegans [12] . Sirtuins are also required for calorie restriction (CR)-induced life span extension in certain genetic backgrounds [13] , [14] . CR is the only dietary regimen that delays ageing and promotes life span extension in a wide variety of organisms. For example, an increase in Drosophila Sir2 (dSir2) extends their life span, while a decrease in dSir2 shortens it and also blocks the life span extension induced by CR [13] , [15] . Moreover, the overexpression of dSir2 in the fat body, but not in muscles, leads to a longevity phenotype in Drosophila under a standard diet (2.5% yeast), but not under a yeast-restricted diet (0.25% yeast). In this case, the levels of dSir2 overexpression are comparable to those induced by a yeast-restricted diet. These results suggest that dSir2 in the fat body regulates life span in a diet-dependent manner [16] . Although one study failed to show life span extension in dSir2-overexpressing flies [2] , this might be due to an excessive amount of dSir2 out of an optimal range for life span extension. In fact, the effect of dSir2 on life span is dose-dependent, and two- to fivefold increases in dSir2 are suitable to promote life span extension, whereas higher levels of dSirt2 decrease life span [15] . Taken together, these recent studies clearly reaffirm that sirtuins function as an evolutionarily conserved regulator of ageing and longevity in these model organisms. An important question still remains: do sirtuins play a role in the regulation of ageing and longevity in mammals, as they do in other organisms? The mammalian Sir2 orthologue Sirt1 is critical to regulate CR-induced phenotypes in mammals. Whereas knocking out Sirt1 throughout the body or specifically in the brain of mice abrogates the response to CR [14] , [17] , [18] , Sirt1 -overexpressing transgenic mice display CR-mimicking phenotypes [14] or preventative effects of metabolic complications induced by a high-fat diet and ageing [19] , [20] . These results provided a hope to see Sirt1-dependent life span extension in mice. Nonetheless, survival curves of transgenic mice overexpressing Sirt1 (up to threefold) throughout the body and their wild-type controls have been reported to be indistinguishable for both males and females [1] , although these transgenic mice exhibit anti-ageing phenotypes, including lower levels of DNA damage and spontaneous cancer incidence, better glucose tolerance, higher bone density and lower levels of p16 lnk4a , a well-established marker of ageing [1] , compared with wild-type mice. Remarkably, we have recently demonstrated that mice with brain-specific overexpression of Sirt1 show a significant delay in ageing and extension of their life span in both males and females (see below) [3] . In addition, transgenic males overexpressing Sirt6 show a significantly longer life span compared with control males [21] . They also display better glucose tolerance, lower serum levels of insulin-like growth factor 1 (IGF-1), higher levels of IGF-binding protein 1 and lower phosphorylation levels of Akt, Foxo1 and Foxo3, major components of IGF-1 signalling, in white adipose tissue (WAT). This life span extension observed in Sirt6 -transgenic males might be partially due to a protective role of Sirt6 against lung cancer. In these transgenic mice, Sirt6 is also ectopically overexpressed, potentially causing some non-physiological effects. Therefore, more mechanistic details need to be carefully addressed for this Sirt6-driven life span extension [21] . In humans, analyses of Sirt3 polymorphisms in a large population of individuals at 20–106 years of age implicate a direct link between Sirt3 and longevity [22] , [23] . Further study will be desirable to determine whether mice with overexpressing Sirt3 could extend life span. Finally, several lines of evidence implicate the involvement of Sirt7 in age-associated pathophysiology. Sirt7 -deficient mice show a shortened life span with enhanced cardiomyopathy compared with controls [5] , [6] , and knocking out Sirt7 in cells induces apoptosis, suggesting that Sirt7 is required for cell survival [5] , [6] . Taken together, there are now increasing lines of evidence strongly suggesting that sirtuins play an important role in delaying the ageing process and promoting longevity in mammals. Recent studies have revealed the importance of sirtuins in the brain for ageing and longevity control in mammals. Particularly, hypothalamic sirtuins govern multiple physiological functions, including feeding behaviour, endocrine regulation, physiological rhythms and emotion ( Table 1 ). These hypothalamic functions decline with advanced age, influencing the ageing process and longevity (see below). Most studies have focused on the function of Sirt1; therefore, we will mainly focus on the function of Sirt1 in the hypothalamus ( Fig. 1 ). The function of Sirt1 in other brain regions and the functions of other sirtuins in the brain will briefly be discussed in the context of their roles in ageing. Figure 1: Schematic diagrams of brain sections. Sections represent the approximate posterior levels to Bregma −0.58 mm ( a ), −1.70 mm ( b ) and −2.30 mm ( c ). The locations of the hypothalamic nuclei are indicated by the following: LH, lateral hypothalamus; PVN, paraventricular nucleus; SCN, suprachiasmatic nucleus; DMH, dorsomedial hypothalamus; VMH, ventromedial hypothalamus; Arc, arcuate nucleus; PH, posterior hypothalamus. Images adapted, with permission, from Franklin, K.B.J. & Paxinos, G. The Mouse Brain in Stereotaxic Coordinates 2nd edn, copyright Academic Press (2001). Full size image Feeding behaviour The role of hypothalamic Sirt1 in feeding behaviour has been studied extensively; however, the results are varied between experimental approaches. Feeding behaviour is controlled by the neuronal circuit through hypothalamic nuclei, particularly through the arcuate, lateral and paraventricular nuclei of the hypothalamus (Arc, LH and PVN, respectively). This neuronal circuit comprises orexigenic neurons containing neuropeptide Y (Npy)/agouti-related peptide (Agrp) or orexin/hypocretin (Hcrt), and anorexigenic neurons containing proopiomelanocortin (Pomc)/cocaine and amphetamine-regulated transcript (Cart). Among those hypothalamic nuclei, the Arc has a high sensitivity to peripheral signals such as hormones and cytokines due to its position adjacent to the medial eminence and serves as an interface between the neural and peripheral endocrine systems. Intracerebroventricular (icv) administration of EX527, a Sirt1 selective inhibitor, into the Arc or knockdown of Sirt1 by small interfering RNA in the Arc inhibits food intake in rodents by reducing the level of Agrp and increasing the level of Pomc [24] . On the other hand, mice with deletion of Sirt1 specifically in the Pomc neurons are more susceptible to diet-induced obesity; however, these mice show indistinguishable food intake compared with control mice [25] . In addition, icv administration of Sirt1 -expressing adenovirus into the mediobasal hypothalamus (MBH) also suppresses feeding behaviour [26] . Other in vitro studies indicate that Sirt1 regulates the transcription of anorexigenic/orexigenic neuropeptides. Sirt1 suppresses Foxo1-induced Agrp promoter activity in HEK293 cells [26] . Foxo1 upregulates the transcription of Npy and Agrp in cultured cell lines, and hypothalamic Foxo1 controls food intake in vivo [27] , [28] . The regulation of Pomc promoter activity by Sirt1 still remains undetermined [24] , [26] . Given these contradictory results, the mechanisms by which hypothalamic Sirt1 controls feeding behaviour through modulating hypothalamic orexigenic and/or anorexigenic neuropeptides need to be further elucidated by using mouse models with neuron-specific genetic manipulation. Sirt1 is also required to mediate the orexigenic action of ghrelin, a stomach-derived peptide that increases food intake through the activation of hypothalamic AMP-activated protein kinase (AMPK). The icv administration of EX527 blunts the ghrelin-induced food intake in rats [29] , and mice with deletion of p53, a target of Sirt1, fail to respond to ghrelin in feeding behaviour [30] . Nonetheless, given that the central administration of Aminoimidazole-4-carboxamide ribonucleotide (AICAR), a potent AMPK activator, is still able to increase food intake in p53- knockout mice, p53 is not required for the orexigenic action of direct AMPK activators, and the hypothalamic Sirt1/p53 pathway is likely to be specific for mediating the orexigenic action of ghrelin [30] . Interestingly, the icv injection of ghrelin increases food intake in a dose-dependent manner in young Wister rats, whereas the effect of ghrelin-induced food intake is reduced with advanced age [31] . Most effects of ghrelin are exerted through the growth hormone (GH) secretagogue receptor, which is a receptor for ghrelin and is expressed in hypothalamic neurons including Npy/Agrp neurons [32] . Therefore, Sirt1 might regulate ghrelin-induced food intake by modulating the function of Npy/Agrp neurons. Given that Sirt1 activity decreases in peripheral tissues over age due to decreases in NAD + (ref. 33 ), a similar event might occur in the hypothalamus, potentially resulting in the decrease in food intake during ageing [34] , [35] . If this is the case, maintaining Sirt1 activity in the hypothalamus could be an effective therapeutic intervention to prevent anorexia in the elderly. Endocrine regulation Sirt1 regulates the hypothalamic–pituitary axis by the synthesis and secretion of hormones in the hypothalamus and pituitary gland. The hypothalamus controls various endocrine systems through synthesizing and secreting specific hormones that stimulate or inhibit the secretion of pituitary hormones controlling many physiological processes. For example, Sirt1, Foxo1 and necdin, a versatile protein to promote differentiation and survival of mammalian neurons, are co-expressed in Arc neurons and have been reported to control thyroid function [36] . In the hypothalamic–pituitary–thyroid axis, the thyroid gland secretes triiodothyronine (T 3 ) and tetraiodothyronine (T 4 ) in response to thyroid-stimulating hormone (TSH) produced in the anterior pituitary gland. TSH is secreted in response to thyroid-releasing hormone (TRH) synthesized and secreted by neurons in the PVN. In Necdin- knockout mice, the expression of Npy/Agrp in the hypothalamus is upregulated, whereas levels of TRH mRNA in the PVN, hypothalamic proTRH protein and serum TSH, T 3 and T 4 are all significantly reduced. Indeed, Necdin, Foxo1 and Sirt1 are found to bind to the Agrp promoter. These results indicate that Sirt1 suppresses Npy/Agrp expression in the Arc and directly increases TRH production and secretion in the PVN, resulting in activation of the hypothalamic–pituitary–thyroid axis. Another example is the regulation of the hypothalamic–pituitary–gonadal axis by Sirt1. Gonadotropin-releasing hormone (Gnrh) is a hormone mainly generated and secreted from the hypothalamus that stimulates the secretion of pituitary gonadotropins (follicle-stimulating hormone and luteinizing hormone), promoting the production of sex hormones (testosterone and oestrogen). Sirt1- knockout mice on the 129/SV background display a significant reduction in Gnrh expression in the hypothalamus and arrested spermatogenesis before the completion of meiosis [37] . Similarly, defective phenotypes of spermatogenesis are observed in Sirt1- knockout mice on CD-129/SV and C57BL6 backgrounds [38] , [39] . Future investigations should address whether the reduction of Gnrh in the hypothalamus is a direct result of changes in hypothalamic Sirt1. Sirt1 is also abundantly expressed in the pituitary gland and regulates pituitary hormone secretion and/or synthesis, such as TSH [40] and GH [17] , [41] . A number of papers report that very complex changes occur in endocrine systems during the ageing process in mammals [42] . Dissecting the age-associated alterations of Sirt1 function in hypothalamic nuclei and pituitary gland will provide a great perspective on the importance of the endocrine system in governing mammalian ageing and longevity. Although hypothalamic sirtuins might regulate the hypothalamus–pituitary axis for GH/IGF-1 signalling, the mechanism remains undetermined. IGF-1 is secreted mainly from the liver in response to GH that is secreted from the anterior pituitary gland. GH secretion is regulated by GH-releasing hormone(Ghrh) that is mainly generated and secreted from the Arc of the hypothalamus. Neuron-specific Sirt1 -knockout mice, which show efficient deletion of Sirt1 in the brain but not in other tissues such as pituitary gland, display lower levels of GH and IGF-1 (refs 17 , 41 ). Similarly, neuron-specific Sirt6- knockout mice display reduced GH and IGF-1 levels without altering Ghrh expression in the hypothalamus [43] . This finding suggests the possibility that the feedback mechanism to the hypothalamus is dysfunctional in Sirt1- and Sirt6- knockout mice. On the other hand, Sirt6- overexpressing transgenic mice also show reduced serum levels of IGF-1 (ref. 21 ). As GH/IGF-1 signalling is one of the key longevity pathways, exploring the role of hypothalamic Sirt1 and Sirt6 in the GH/IGF-1 signalling pathway will provide better understanding of hormone-dependent ageing and longevity control in mammals (see also the section ‘Systemic regulation of ageing and longevity by brain sirtuins’). Physiological rhythms A recent study has demonstrated that Sirt1 mediates central circadian control in the suprachiasmatic nucleus (SCN) of the hypothalamus. As a circadian pacemaker, neurons in the SCN regulate physiological homeostasis such as physical activity, endocrine system, body temperature, feeding behaviour and the sleep and wake cycle through clock regulators such as Clock, Bmal, Per and Cry. Brain-specific Sirt1- overexpressing transgenic mice show decreases in the level of acetylated Bmal1 in the SCN, whereas brain-specific Sirt1- knockout mice show increases in its acetylation [44] . Sirt1 directly activates Bmal1 transcription, which is positively regulated by the nuclear receptor RORα, and this activation requires PGC-1α, a key Sirt1 target [44] . In addition, the protein levels of Sirt1 decrease in the SCN with advanced age, as do the levels of Bmal1 and Per2 proteins. Moreover, ageing reduces the ability to adapt to an abrupt change in the light/dark cycle (for example, jet lag), causing the deficit in circadian regulation, and mice maintaining a circadian period close to 24 h live longer than mice with circadian period significantly longer or shorter than 24 h [45] . Interestingly, young mice lacking Sirt1 in the brain phenocopy these age-dependent circadian changes, whereas mice overexpressing Sirt1 in the brain are protected from such effects of ageing [44] . These results indicate that maintaining Sirt1 function in the SCN could delay the ageing process and promote life span extension, although a study using transgenic mice with SCN-specific manipulation of Sirt1 will be necessary to address this possibility. Hypothalamic Sirt1 is also involved in the regulation of food-entrained behavioural rhythms. As food is one of the critical cues to integrate diurnal physiological rhythms in mammals, rodents alter their physiological functions, such as physical activity, body temperature and arousal in response to changes in food availability. These food-entrained behavioural rhythms are a well-established experimental model to study circadian physiological rhythms. Brain-specific Sirt1- overexpressing transgenic mice, called BRASTO mice, exhibit significant enhancement of food-anticipatory activity, whereas Sirt1- knockout mice abrogate this activity [18] . In this model, the dorsomedial hypothalamus (DMH), especially the compact region of the DMH, plays an important role in the regulation of food-entrained behavioural rhythms [46] , although some controversy remains [47] . A recent study demonstrated that scheduled feeding induces neural activation in the Arc and DMH [48] . Analysis of phosphorylated ribosomes immunoprecipitated from mouse hypothalami, which they describe as a novel method to capture and analyse activated neurons, identified genes including pro-FMRFamide-related neuropeptide VF (Npvf), prodynorphin (Pdyn), GP50 and G-substrate gene (Gsbs) as highly expressed genes in activated DMH neurons under food-entrained circadian rhythm [48] . BRASTO mice show increases in neuronal activity in the DMH and LH under scheduled feeding, whereas Sirt1- knockout mice show significant decreases in neuronal activity in the DMH and LH, suggesting that Sirt1 in the DMH and LH plays a crucial role in the regulation of food-entrained behavioural rhythms by enhancing neuronal activity in the DMH and LH [18] . Whether activated neurons in the DMH of BRASTO mice also express Npvf , Pdyn , GP50 and/or Gsbs , is still unknown. It will be of great interest to address whether Sirt1 modulates expressions of these genes, as well as other important genes, in the DMH. In addition, the food-anticipatory activity is similar in rats at 11 weeks and 9 months of age; however, this activity is significantly reduced in rats at 12 and 24 months of age [49] , suggesting the age-associated circadian deficit in this paradigm as well as in the jet-lag paradigm. Therefore, these findings also provide further support to the notion that maintaining Sirt1 function in the hypothalamus, particularly the DMH and LH, can probably counteract age-associated pathophysiological changes and contribute to extension of life span [3] . Although it is not clear whether hypothalamic Sirt1 controls the sleep and wake cycle through circadian regulation, Sirt1 in the hypothalamus seems involved in the homeostatic regulation of sleep. Sleep and wake cycle is controlled by circadian and homeostatic factors. Mice with knockdown of Sirt1 in the DMH/LH have significantly decreased quality of sleep [3] . A number of studies demonstrate that quality of sleep declines with age, as determined by the quantity of delta activity (delta power) in the electroencephalogram during non-rapid eye movement sleep [50] . In addition, human aetiological studies show a correlation between non-rapid eye movement delta power and life span, and an inverse correlation with metabolic complications [51] . However, the molecular mechanisms behind these phenomena are not fully understood. Interestingly, it has been reported that Sirt1 exists in wake-active neurons, and is necessary for neurotransmitter synthesis of wake-active neurons [52] . Conditional whole-brain Sirt1 -knockout mice display a reduction of wake time in both light and dark periods. Furthermore, Sirt1- deficient mice develop an accelerated accumulation of lipofuscin, a fluorescent pigment accumulating with age, in the cytoplasm of cells of the central nervous system. The connection between sleep and wake regulation and ageing and longevity control has been poorly understood in mammals. Therefore, elucidating the function of hypothalamic Sirt1-positive neurons in sleep and wake regulation will probably shed new light onto this fascinating connection. Emotion Brain sirtuin also regulates mood and behaviour [53] . Studies using brain-specific gain- and loss-of-function mouse models of Sirt1 have demonstrated that upregulation of Sirt1 leads to anxiety drive by activating the transcription of the gene encoding monoamine oxidase-A, an enzyme that deaminates neurotransmitters such as serotonin. Monoamine oxidase inhibitors are clinically applied for depression and anxiety patients [54] . In addition, both common and rare variants in Sirt1 have been found to be associated with anxiety and other psychiatric disorders [53] . In the hypothalamus, the LH plays an important role in the regulation of reward and motivation, and orexin/Hcrt has only recently been identified as a key neurotransmitter involved in this function [55] . Orexin/Hcrt is mainly expressed in the hypothalamus, especially in the LH [56] . Orexin/Hcrt neurons project to the amygdala, the integrative centre for emotions, emotional behaviour and motivation. As the number of orexin/Hcrt neurons and their activity decline with age in rats [57] , [58] and orexin-A-labelled neurons are all Sirt1- positive in B6 male mice [52] , this age-related reduction of orexin/Hcrt-neuronal function could influence age-associated changes in emotion and motivation possibly through Sirt1 function. Orexin neuron-specific Sirt1- knockout or -overexpressing mice would be crucial models to understand the physiological importance of Sirt1 in the regulation of emotion. Further evidence suggesting that sirtuins regulate behaviour is that orexin/Hcrt neurons have anatomical connections with reward-associated brain regions including nucleus accumbens (NAc) and ventral tegmental area, and Sirt1 and Sirt2 in the NAc regulate behavioural responses to cocaine and morphine [59] . Mice overexpressing Sirt1 or Sirt2 in the NAc enhance the rewarding behaviours in response to cocaine and morphine, whereas NAc-specific Sirt1- knockdown mice decrease this drug-rewarding behaviour. The LH also has an anatomical connection to the anterior cigulate cortex, a key area that functions as an interface between emotion and cognition [60] , and regulates emotional experiences in ageing [61] . Exploring such a new possibility that neural circuits between LH orexin neurons, Sirt1/Sirt2-positive neurons in NAc and anterior cigulate cortex neurons regulate the emotional experience might expand potential clinical applications of sirtuin-targeting therapeutics to treat age-associated emotional disorders. Brain plasticity Brain sirtuins modulate the capacity of the nervous system to change neuronal structure and functions. For example, Sirt1 regulates synaptic plasticity [29] , [62] , [63] , including long-term potentiation [62] , neuronal ultrastructure [52] and neurogenesis [64] , [65] , [66] , and ultimately influences learning and memory [62] , [67] . In addition, large bodies of evidence indicate that brain Sirt1 has neuroprotective effects against age-associated neurological disorders such as Alzheimer’s disease, Parkinson’s disease, Huntington’s disease and amyotrophic lateral sclerosis [4] , [67] . Contrarily, inhibiting Sirt2 reduces α-synuclein toxicity and modifies inclusion morphology in a cellular model of Parkinson’s disease [68] . Overexpression of Sirt3 inhibits mitochondrial reactive oxygen species production in mouse primary cerebral cortical neurons, whereas knockdown of Sirt3 enhances excitotoxic neuronal death, suggesting that Sirt3 can protect against excitotoxic injury [69] . These findings highlight the benefits of manipulating sirtuin activity to preserve brain function and prevent age-associated neurological disorders. As discussed above, sirtuins are clearly important for various hypothalamic and brain functions, and their functions appear to be reduced during the ageing process, potentially causing age-associated deficits in these hypothalamic/brain functions. However, does it mean that brain sirtuins are indeed capable of modulating ageing and longevity in mammals? The answer to this critical question appears to be yes. So far, an accumulating body of evidence has pointed out the importance of the hypothalamus in controlling mammalian longevity [3] , [70] , and also suggested the involvement of hypothalamic sirtuins, especially Sirt1, in this regulation. DMH and LH We have recently demonstrated that increasing Sirt1 in the hypothalamus, particularly in the DMH and LH, delays ageing and extends life span [3] ( Fig. 2 ). In our previous study, we demonstrated that BRASTO mice show enhanced physiological responses to diet-restricted conditions through the upregulation of Ox2r expression [18] , an important downstream target gene of Sirt1 in the hypothalamus. Thus, we hypothesized that BRASTO mice might live longer than control mice. Strikingly, BRASTO mice extend median and maximal life span in both males and females. Associated with this life span extension, several physiological phenotypes of BRASTO mice, including physical activity, body temperature, O 2 consumption and quality of sleep, are significantly maintained during the ageing process. Particularly, their skeletal muscle maintains youthful morphology and function of the mitochondria during the ageing process due to enhanced sympathetic nervous tone during the dark period. This phenotype results from enhanced neural activity in the DMH and LH during the dark period in aged BRASTO mice, through the upregulation of Ox2r expression by Sirt1 and its novel partner Nkx2-1, an Nk2 family homeodomain transcription factor, in these hypothalamic nuclei. Although the mechanism by which the signal from the hypothalamus is specifically directed to skeletal muscle still remains unknown, it is possible that skeletal muscle stimulated by the sympathetic nervous system leads to systemic events that contribute to the delay in ageing and life span extension. A study by DMH/LH-specific Sirt1 , Nkx2-1 and Ox2r knockdown further demonstrated the importance of Sirt1/Nkx2-1/Ox2r-mediated signalling pathway to counteract age-associated physiological decline. Furthermore, stereotactic injection of Sirt1 -expressing lentiviruses into the DMH of aged wild-type mice ameliorates age-associated declines in physical activity and body temperature, further supporting the notion that the hypothalamus, especially the DMH and LH, is one of the control centres for mammalian ageing and longevity [3] . In the DMH and LH, Sirt1 and Nkx2-1 are highly colocalized in a specific subset of neurons. These novel Sirt1/Nkx2-1 double-positive neurons must be key to modulate systemic ageing and possibly life span in mammals. The precise characterization of these Sirt1/Nkx2-1 double-positive neurons in the DMH and LH is currently in progress. 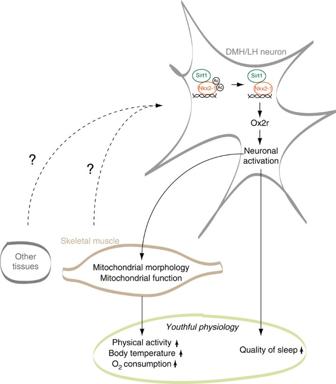Figure 2: Sirt1/Nkx2-1/Ox2r-mediated signalling in DMH and LH neurons systemically regulates ageing/longevity in mammals. In the dorsomedial and lateral hypothalamic nuclei (DMH and LH, respectively), Sirt1 interacts with and deacetylates Nk2 homeobox 1 (Nkx2-1), increasesorexin type 2 receptor (Ox2r)transcription and enhances neural activation. The neural activation of the DMH and LH guides skeletal muscle to maintain mitochondrial morphology and function through sympathetic nervous tones. Sustaining DMH/LH function during the ageing process leads to preserved youthful physiology, including physical activity, body temperature, oxygen consumption and quality of sleep. The crosstalk between the hypothalamus and skeletal muscle might be critical to regulate systemic ageing, although this possibility is currently under investigation. Figure 2: Sirt1/Nkx2-1/Ox2r-mediated signalling in DMH and LH neurons systemically regulates ageing/longevity in mammals. In the dorsomedial and lateral hypothalamic nuclei (DMH and LH, respectively), Sirt1 interacts with and deacetylates Nk2 homeobox 1 (Nkx2-1), increases orexin type 2 receptor (Ox2r) transcription and enhances neural activation. The neural activation of the DMH and LH guides skeletal muscle to maintain mitochondrial morphology and function through sympathetic nervous tones. Sustaining DMH/LH function during the ageing process leads to preserved youthful physiology, including physical activity, body temperature, oxygen consumption and quality of sleep. The crosstalk between the hypothalamus and skeletal muscle might be critical to regulate systemic ageing, although this possibility is currently under investigation. Full size image Interestingly, we had another independent line of BRASTO mice, which showed much higher Sirt1 expression through the hypothalamus, but not DMH/LH predominantly. Surprisingly, this particular line exhibited the complete lack of life span extension and beneficial physiological phenotypes during the ageing process. The Arc in those transgenic mice showed much higher neural activity during the dark time compared with controls, whereas no enhancement of neural activity was observed in the DMH and LH. Therefore, the Arc neurons might have certain suppressive effects on the function of the DMH/LH neurons, comprising a neural circuit that controls ageing and longevity in mammals. In such a neural circuit between the Arc and DMH/LH, the balance of their neural activities might be a critical determinant for delayed ageing and life span extension. This idea could potentially provide a testable explanation as to why previously generated whole-body Sirt1 -overexpressing transgenic mice failed to show life span extension. Those whole-body Sirt1 overexpressors might have high Sirt1 expression through all hypothalamic nuclei, suppressing the functional dominance of the DMH and LH. To further test this idea, it will be of great importance to manipulate Sirt1 dosage in each hypothalamic nuclei and examine what happens to age-associated pathophysiology and eventually life span in those mice. Arc and ventromedial hypothalamus Although we still do not know whether the balance of neural activities between hypothalamic nuclei might be a critical determinant for delayed ageing and life span extension, the roles of Sirt1 in other hypothalamic nuclei, such as the Arc and ventromedial hypothalamus (VMH), have been studied, at least for the regulation of energy metabolism. For example, Sirt1 in Pomc neurons, which belong to the central melanocortin system and reside in the Arc and hindbrain nucleus of the solitary tract, is required for homeostatic defenses against diet-induced obesity [25] . Mice lacking Sirt1 in Pomc neurons show decreases in O 2 consumption and heat production due to the impairment of brown adipose tissue (BAT)-like remodelling of perigonadal WAT under a high-calorie diet. In addition, mice lacking Sirt1 in steroidogenic factor 1 (SF1) neurons, which are unique cells in the VMH, show higher susceptibility to diet-induced type 2 diabetes due to impaired insulin sensitivity in skeletal muscle compared with control mice [71] . Under a high-calorie diet, SF1 neuron-specific Sirt1- knockout mice show impaired glucose tolerance, insulin resistance, increases in body weight, fat mass, blood glucose, serum leptin and serum insulin, and decreases in O 2 consumption, CO 2 production and ambulatory movements. Furthermore, Sirt1 in SF1 neurons is required for the normal metabolic action of orexin-A [71] . Increasing Sirt1 in SF1 neurons protects against high-fat diet-induced glucose and insulin imbalances by enhancing muscle insulin sensitivity, further supporting the notion that Sirt1 in the VMH regulates signals to skeletal muscle and maintains its insulin sensitivity. Other studies also provide compelling evidence for the importance of brain Sirt1 in the systemic regulation of glucose and lipid metabolism, although the direction of its effect is sometimes contradictory [63] , [72] . All these studies point out that Sirt1 function is crucial in the Arc, VMH and other brain regions for the systemic regulation of energy metabolism. Nonetheless, it has still been poorly understood how exactly such regulation is coordinated through multiple hypothalamic or brain regions. For example, the BAT-like remodelling, which is regulated by Sirt1 in the Pomc neurons in mice [25] , is also regulated by Npy neurons in the DMH in rats [73] . Rats with adeno-associated virus-mediated knockdown of Npy in the DMH show decreases in inguinal fat weight under a regular diet, and ameliorates high-fat diet-induced obesity by the development of BAT within WAT and activation of the BAT through sympathetic nerve stimulation [73] . Although it is not clear whether this regulation is species-specific, it is likely that increasing Sirt1 activity in the Arc, which mostly results in metabolic benefits at a systemic level, could modulate neural activities in other hypothalamic nuclei, such as the DMH and LH, and affect the ageing process and eventually longevity. If this is the case, the gain of metabolic benefits, such as enhanced insulin sensitivity, might not always be associated with delay in ageing and longevity, dependent on how neural activities in each hypothalamic nucleus and other brain regions are coordinated. Mediobasal hypothalamus To achieve such complex coordination of neural activities in different regions, sirtuins must cooperate with other key regulators and signalling pathways in hypothalamic neurons and even in other cell types in the brain. The MBH regulates mammalian ageing and longevity through modulating immune responses and endocrine systems during the ageing process [70] . The MBH is the most sensitive region to nuclear factor-κB (NF-κB) activation during the ageing process compared with other brain regions such as the cortex and hippocampus. NF-κB activation is a stress signal pathway that stimulates immune responses. Remarkably, MBH-specific injection of dominant-negative IκB-α to inhibit NF-κB in MBH neurons prolongs life span, whereas MBH-specific injection of constitutively active IKK-β to activate NF-κB in MBH neurons shortens life span. These findings suggest that attenuation of NF-κB activity in the hypothalamus is critical to control mammalian longevity. Interestingly, icv or subcutaneous administration of GnRH prevents the age-associated decline in neurogenesis in the hypothalamus and hippocampus, muscle strength (endurance), muscle (fibre) size, skin thickness, bone mass and tail tendon collagen integrity. Indeed, transcription of the Gnrh gene in the hypothalamus declines as a result of NF-κB activation over age. Compared with hypothalamic neurons showing NF-κB activation at a later stage of ageing, NF-κB activation in microglia is observed at an earlier stage of ageing, coupled with tumour necrosis factor-α generation. It appears that microglial NF-κB activation results in the production of tumour necrosis factor-α, which stimulates hypothalamic neurons and activates their NF-κB [74] , possibly causing systemic ageing. Although what triggers microglial NF-κB activation in the MBH during the ageing process needs to be investigated, it is of great interest that Sirt2 functions as an inhibiter of microglia-mediated inflammation and neurotoxicity [75] . Sirt2 -knockout mice display enhanced microglial activation induced by the injection of lipopolysaccharide, a well-established pro-inflammatory stimulus that binds to Toll-like receptor 4 (TLR4) exclusively expressed on microglia in the mouse brain. Stimulation of TLRs in microglia triggers central nervous system inflammation mainly through NF-κB-dependent activation. Knockdown of Sirt2 also exaggerates microglial activation induced by several different stimuli through TLR2, 3 and 4 in cultured microglial cell lines [75] . These findings imply the possibility that age-associated decline in Sirt2 activity triggers NF-κB activation in microglia in the MBH, possibly leading to neural NF-κB activation ( Fig. 3 ). 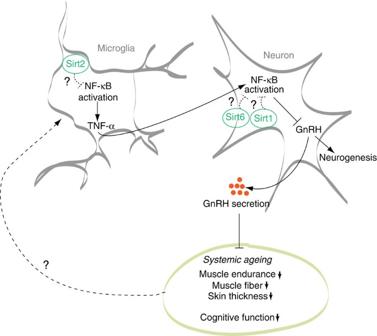Figure 3: NF-κB signalling in the MBH systemically regulates mammalian ageing and longevity. In the MBH, NF-κB activation in microglial cells enhances the production and secretion of the inflammatory cytokine tumour necrosis factor (TNF)-α, leading to the activation of NF-κB in Gnrh neurons. Circulating Gnrh influences systemic ageing phenotypes, including muscle endurance, the size of muscle fibre and skin thickness as well as cognitive functions. Supplementation of Gnrh into the brain also upregulates neurogenesis. Sirt1 and Sirt2 might function as an inhibitor of NF-κB activity in the neurons and/or microglia of the MBH during the ageing process. Figure 3: NF-κB signalling in the MBH systemically regulates mammalian ageing and longevity. In the MBH, NF-κB activation in microglial cells enhances the production and secretion of the inflammatory cytokine tumour necrosis factor (TNF)-α, leading to the activation of NF-κB in Gnrh neurons. Circulating Gnrh influences systemic ageing phenotypes, including muscle endurance, the size of muscle fibre and skin thickness as well as cognitive functions. Supplementation of Gnrh into the brain also upregulates neurogenesis. Sirt1 and Sirt2 might function as an inhibitor of NF-κB activity in the neurons and/or microglia of the MBH during the ageing process. Full size image On the other hand, other sirtuins, Sirt1 and Sirt6 in particular, might also be involved in the regulation of NF-κB activation in neurons during ageing. It has been known that Sirt1 deacetylates the p65 subunit of NF-κB and suppresses the transcriptional activity of NF-κB [76] . Sirt6 also attenuates NF-κB signalling by deacetylating lysine 9 of histone H3 at NF-κB target loci, inhibiting apoptosis and cellular senescence [77] . Therefore, Sirt1 and Sirt6 might be crucial to control NF-κB signalling in neurons, whereas Sirt2 does so in microglia. It appears that all these sirtuin activities decrease over age, all contributing to the activation of NF-κB signalling. It will be very interesting to examine whether NAD availability declines in all or specific hypothalamic nuclei during the ageing process. Other hypothalamic areas Similar to Sirt1, the role of Sirt6 in the hypothalamus could be multifaceted. As discussed in the previous section, there is an interesting but underinvestigated connection between Sirt6 and GH/IGF-1 signalling. Mice homozygous for the Ghrh receptor gene show decreases in plasma GH levels and reveal longer life span in both males and females compared with heterozygous controls [78] . In addition, Ghrh- knockout mice show robust increases in median and maximum life span in both males and females [79] . Ghrh- knockout mice exhibit lower levels of body weight, fasted blood glucose, insulin, IGF-1 and the homeostatic model assessment index, improved insulin tolerance, higher respiratory quotient and major shifts in gene expression profiles related to xenobiotic detoxification, stress resistance and insulin signalling in the liver. Interestingly, there is a significant overlap between genes affected by the knockout of Ghrh and the overexpression of fibroblast growth factor 21 (Fgf21) [79] . FGF21 is a hepatokine that plays a role in eliciting and coordinating the adaptive starvation response. Fgf21 -overexpressing transgenic mice show life span extension [80] , and recent studies demonstrate the connection between FGF21 and hypothalamic functions [81] , [82] . These findings lead to a speculation that FGF21 functions to modulate hypothalamic Ghrh neurons that could be potentially regulated by hypothalamic Sirt1 and/or Sirt6 ( Fig. 4 ). It will be of great interest to examine whether Sirt1 and/or Sirt6 are indeed necessary for the regulation of hypothalamic Ghrh neuronal activity. Taken together, sirtuins in the brain, the hypothalamus in particular, play important roles in coordinating complex neural activities and modulating the ageing process and longevity in mammals. 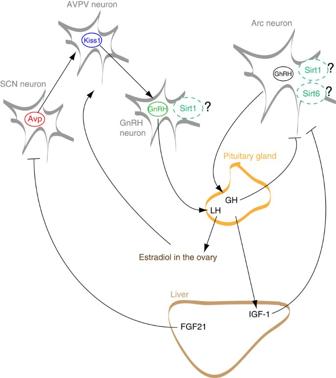Figure 4: GH/IGF-1 signalling in the systemic regulation of mammalian longevity. Ghrh is secreted from neurons in the Arc and stimulates GH secretion from somatotropic cells of the anterior pituitary gland. The GH leads to secretion of IGF-1 from the liver. GH and IGF-1 have a negative feedback to the hypothalamus for the regulation of Ghrh production/secretion. Gnrh is secreted from neurons in the Arc and stimulates luteinizing hormone (LH) secretion from gonadotroph cells in the anterior pituitary gland. FGF21, a hepatokine that can promote longevity in mice, enters into the brain and acts on the SCN neurons to suppress vasopressin (Avp) that enhancesKiss1expression in the anteroventral periventricular nucleus of the hypothalamus (AVPV). AVPV neurons stimulate Gnrh neurons that regulate gonadotropin secretion in the pituitary, and receive a positive feedback from the circulating estradiol. Sirt1 and Sirt6 might regulate the function of Gnrh and Ghrh neurons, respectively, in the hypothalamus. Figure 4: GH/IGF-1 signalling in the systemic regulation of mammalian longevity. Ghrh is secreted from neurons in the Arc and stimulates GH secretion from somatotropic cells of the anterior pituitary gland. The GH leads to secretion of IGF-1 from the liver. GH and IGF-1 have a negative feedback to the hypothalamus for the regulation of Ghrh production/secretion. Gnrh is secreted from neurons in the Arc and stimulates luteinizing hormone (LH) secretion from gonadotroph cells in the anterior pituitary gland. FGF21, a hepatokine that can promote longevity in mice, enters into the brain and acts on the SCN neurons to suppress vasopressin (Avp) that enhances Kiss1 expression in the anteroventral periventricular nucleus of the hypothalamus (AVPV). AVPV neurons stimulate Gnrh neurons that regulate gonadotropin secretion in the pituitary, and receive a positive feedback from the circulating estradiol. Sirt1 and Sirt6 might regulate the function of Gnrh and Ghrh neurons, respectively, in the hypothalamus. Full size image As brain sirtuins, Sirt1 in particular, regulate many important pathophysiological aspects of ageing, modulating brain sirtuin activity could be an effective preventive/therapeutic intervention to slow down ageing and extend at least health span. Until now, a number of small-molecule chemical activators of Sirt1 have been identified. Resveratrol, a natural polyphenolic compound found in grapes and other plants, is one of these sirtuin-activating compounds (STACs). Interestingly, resveratrol has been proven to show beneficial effects of treating age-associated diseases including Alzheimer’s disease, Parkinson’s disease, Huntington’s disease, amyotrophic lateral sclerosis, stroke and cognitive deficits [83] , [84] . In addition, administration of resveratrol also ameliorates diet-induced metabolic complications in mice [5] , but does not show much effects in regular chow-fed rodents [85] . Similar trends have also been observed in human subjects [86] . On the other hand, resveratrol also directly targets proteins other than Sirt1, such as AMPK and cAMP phosphodiesterases [5] . Subsequently, synthetic STACs that are more potent than natural compounds have been developed [87] . These new STACs show beneficial effects on diet-induced metabolic complications [87] and life span extension under a normal diet or a high-fat diet condition [88] . Although the mechanism of STAC action had been controversial [87] , a recent study has provided compelling evidence for the direct activation of Sirt1 by STACs through an allosteric mechanism [89] . STACs bind to an allosteric site, which is a glutamate residue at position 230 (Glu230) that is immediately amino-terminal to the catalytic core of Sirt1, facilitating Sirt1 activity. Therefore, STACs look promising to combat against age-associated disorders, including neurodegenerative diseases and metabolic complications. On the other hand, the role of Sirt1 in cancer, a well-established age-associated disease, is contradictory. Sirt1 acts as both a tumour suppressor and a tumour promoter. This contradiction seems to be explained due to the existence and the genetic alterations of p53 (refs 90 , 91 ), a critical tumour suppressor. To clinically apply Sirt1 activators for cancer treatment, the type of cancer and the stage of its development should be carefully assessed. Recently, supplementation of key NAD + intermediates has drawn much attention as an effective intervention to enhance sirtuin activity and treat age-associated pathophysiology. The supplementation of NAD + per se might not be effective due to its adverse effect, severe hyperglycaemia [92] . We have demonstrated that administration of nicotinamide mononucleotide (NMN), a key NAD + intermediate, dramatically treats symptoms of high-fat diet- and ageing-induced type 2 diabetic mouse models [33] . NMN significantly enhances NAD + production and activates Sirt1 in the liver and other tissues, such as pancreatic β-cells. Another NAD + intermediate, nicotinamide riboside (NR), is also capable of conveying similar effects in the liver and skeletal muscle through the activation of Sirt1 and Sirt3 (ref. 93 ). Inhibiting activities of poly(ADP-ribose) polymerases and CD38/157 ectoenzymes can also increase NAD + levels and activate sirtuins [94] , [95] , although potential sides effects of those inhibitors need to be carefully evaluated. Interestingly, NAD + levels significantly decrease in various tissues and organs during ageing [12] , [33] , leading to reduced sirtuin activity. Thus, it will be of great importance to test whether supplementation of NAD + intermediates, such as NMN and NR, could convey anti-ageing effects on various pathophysiological traits. NAD + intermediates could also enhance sirtuin activity in the brain. Recently, the treatment of Tg2576 AD model mice with NR shows an improvement of cognitive performance [96] . It will be interesting to examine whether NAD + intermediates can enhance sirtuin activity in the hypothalamus. Besides using STACs and NAD + intermediates, sirtuins could be activated by modulating other potential regulators and signalling pathways including deleted in breast cancer 1, active regulator of Sirt1, CCAAT/enhancer-binding protein α and cAMP/protein kinase A pathway [5] . Further drug discovery targeting these regulators and signalling pathways also has a potential to open new avenues for modulating sirtuin activity. Beyond the activation of sirtuins, inhibition of sirtuins could also be applied for the treatment of certain diseases. For instance, Sirt2 inhibitors, such as AGK2, have been reported to treat the pathology of Parkinson’s disease [68] and Huntington’s disease [97] . AGK2 treatment rescues α-Synuclein-mediated toxicity and modifies its aggregation in models of Parkinson’s disease [68] . In addition, in some cases, small molecule Sirt2 inhibitors can selectively induce tumour cell death [98] , [99] , [100] . Taken together, therapeutic and preventive drug development targeting sirtuins is a very promising area of research that has great potential to prevent against age-associated neurodegenerative and metabolic disorders, and lead to extension of human health span. Over the past decade, numerous biological functions of mammalian sirtuins in both peripheral and central systems have been discovered. Subsequently, recent studies have clearly demonstrated the importance of brain Sirt1 and possibly Sirt6 as an evolutionarily conserved regulator of the systemic ageing and longevity in mammals. These studies have made significant advancement to our understanding of how the neural network controls ageing and longevity through specific subsets of neurons in the brain and also of what downstream physiological phenotypes are causally associated with longevity. Nonetheless, several critical questions remain. (1) How does the functional decline in hypothalamic sirtuin activity occur during the ageing process? (2) How and where do different members of the sirtuin family cooperate in this systemic regulation? (3) What factors mediate potential feedback loops between the hypothalamus and peripheral organs and tissues for sirtuin-mediated ageing and longevity control in mammals? (4) What are the most critical physiological phenotype(s) associated with longevity? (5) How can sirtuin activity be specifically modified in the hypothalamus and other brain regions? Further investigation will be required to address these problems to advance our understanding of how brain sirtuins regulate physiological robustness during the ageing process and determine mammalian longevity. It will also be of great importance to translate such knowledge to the development of pharmaceutical and nutriceutical sirtuin-targeting anti-ageing interventions. How to cite this article: Satoh, A. et al. Systemic regulation of mammalian ageing and longevity by brain sirtuins. Nat. Commun. 5:4211 doi: 10.1038/ncomms5211 (2014).